Histology and postural change during the growth of the ceratopsian dinosaurPsittacosaurus lujiatunensis A few dinosaurs are inferred to have undergone an ontogenetic shift from quadrupedal-to-bipedal posture, or vice versa, based on skeletal allometry. The basal ceratopsian Psittacosaurus lujiatunensis is considered to have been mainly bipedal as an adult. Here we infer a postural shift in this species based on a novel combination of limb measurements and histological data. The forelimb is strongly negatively allometric relative to the hindlimb, and patterns of vascular canal orientation provide evidence that growth of the hindlimb was particularly rapid during the middle part of ontogeny. Histology also makes it possible to determine the ontogenetic ages of individual specimens, showing that the forelimb-to-hindlimb ratio changed rapidly during the first or second year of life and thereafter decreased gradually. Occurrence of an ontogenetic shift from quadrupedality to bipedality was evidently widespread in dinosaurs, and may even represent the ancestral condition for the entire group. The first dinosaurs were bipeds, but quadrupedality evolved secondarily in at least four groups: giant sauropodomorphs, thyreophorans, derived ornithopods and ceratopsians [1] . However, ontogenetic studies have shown that even some dinosaurs that remained bipedal as adults had quadrupedal offspring [2] , while conversely some dinosaurs that were quadrupedal when mature had bipedal offspring [3] , [4] . The primary evidence for these postural shifts has come from allometric studies showing shortening or lengthening of the forelimbs, relative to the hindlimbs, over the course of ontogeny. However, no study has simultaneously investigated both limb bone allometry and limb bone histology in any dinosaur, even though histological evidence would make it possible to establish the approximate ontogenetic ages of the specimens included in the analysis and therefore address the timing of postural changes. Furthermore, patterns of differential growth should be reflected in the microstructure of the forelimb and hindlimb bones. Histology has considerable potential as a supplement to allometric studies of dinosaurs, and can potentially provide a continuous record of the growth of an individual bone up to the time of an animal’s death. By contrast, measurements of the dimensions of a limb bone offer only a ‘snapshot’ of the size the bone had reached at that time. However, an obstacle limiting this application of histological analysis is the difficulty of obtaining a sufficiently large sample of individuals at different ontogenetic stages whose limb bones can be sectioned. Psittacosaurus is among the most diverse and abundant dinosaurs, known from 10 or more species and >1,000 specimens from the upper Lower Cretaceous of China, Mongolia, Russia and Thailand [5] . It is a basal member of Ceratopsia, a group that subsequently diversified in the northern continents during the Late Cretaceous to produce a species-rich assemblage of large, horned herbivores. Psittacosaurus is widely interpreted as an obligate or at least habitual biped as an adult [6] , [7] , [8] , [9] , [10] , [11] , [12] , and lay phylogenetically near or even within the transition to the obligate quadrupedality that was characteristic of ceratopsids and possibly some of their closest relatives [12] , [13] , [14] . For these reasons, Psittacosaurus is of intense interest from the perspective of dinosaurian postural evolution, and its abundance in the Lower Cretaceous of Asia makes it a natural subject for palaeobiological analyses in which sample size is a factor. In this paper, we analyse the limb proportions and histology of Psittacosaurus based on many hatchling to adult specimens, to determine whether a postural shift took place during the growth of this dinosaur and investigate the ontogenetic timing of any shift that can be inferred. All of the 16 individuals in our sample were collected from the Lujiatun Beds of the Lower Cretaceous Yixian Formation exposed near Lujiatun Village, Beipiao City, Liaoning Province, China. The majority (10 skeletons) are juveniles that were preserved in clusters of individuals apparently representing the same stage of growth. One of these clusters, accessioned as IVPP (Institute of Vertebrate Paleontology & Paleoanthropology, Beijing) V14341, has previously been interpreted [15] as resulting from burial in a volcanic debris flow that killed the animals instantly. Juvenile individuals were selected for analysis from IVPP V14341 and three similar clusters, but only some of the specimens in each cluster were sufficiently well preserved for inclusion in the study. Almost all of the individuals included in this study, including the two from the cluster described by Zhao et al. [15] , are clearly referable to P. lujiatunensis Zhou et al. [16] All of them have narrow prefrontals, an autapomorphy of P. lujiatunensis [5] , [16] . A shallow depression on the jugal is also present in all the individuals in the sample. This feature is uniquely shared by P. lujiatunensis and Psittacosaurus major , the only other Psittacosaurus species known from the Lujiatun Beds. However, P. major has a characteristically narrow skull roof, a trait not evident in any of the specimens in this study. Other aspects of cranial morphology observed in the specimens are consistent with their referral to P. lujiatunensis , based on published diagnoses [5] , [16] . The only possible exception is the largest individual in the sample (IVPP V12617), which was originally described as an adult of Hongshanosaurus houi [17] . However, this specimen differs in important respects from the juvenile holotype of H. houi , and has been more recently referred to P. lujiatunensis [5] , [18] . This conclusion is tentatively accepted in the present study. Allometric analysis of limb bone proportions within this large sample of P. lujiatunensis shows that the bones of the forelimb are negatively allometric relative to those of the hindlimb, and histological evidence reinforces this result by indicating particularly rapid growth of the hindlimb during the middle part of ontogeny. P. lujiatunensis appears to have undergone a shift from quadrupedality towards bipedality during ontogenetic growth, a pattern that may have been widespread among dinosaurs. Dinosaur age profiles One specimen (IVPP V14342) in the data set was unavailable for histological sampling, but for every other individual we took histological sections from the humerus, radius, ulna, femur, tibia and/or fibula. Across all individuals, a total of 41 bones were sectioned. Three of the individuals were from a cluster (IVPP V16902) of very small juveniles, and sectioning their long bones revealed no lines of arrested growth (LAG). Accordingly, they appear to have been hatchlings <1 year old at the time of death, and they probably represent the smallest Psittacosaurus specimens ever reported (femur lengths 22 and 26 mm). The other individuals in the sample were at least 1 year old. Of the six skeletons from the cluster IVPP V14341 ( Fig. 1 ), five were found to be 2 years old whereas the sixth was found to be 3 years old ( Supplementary Fig. S1 ), indicating slight heterogeneity in the ages of the individuals in this apparent social group. Four of the individuals were from another cluster (ELDM, Erlianhaote Dinosaur Museum, V1038, Supplementary Fig. S2 ), and were all found to be 2 years old. All individuals in the data set that were preserved in isolation (rather than as part of a cluster) and could be studied histologically were at least 5 years old and ranged up to 10 years old ( Supplementary Table S1 ), although the single isolated skeleton (IVPP V14342) that could not be studied histologically was close in size to the 3 years old in cluster IVPP V14341. Conversely, all the specimens in clusters that were studied histologically were 3 years old or younger. 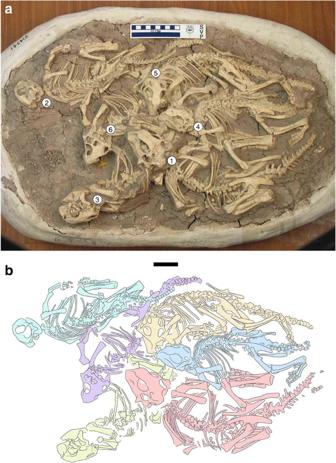Figure 1: Cluster of six juvenilePsittacosaurusfrom the Lower Cretaceous of China. The cluster (IVPP V14341), shown in a photograph (a) and interpretive drawing (b), contains six aligned juvenile specimens ofP. lujiatunensis. Bone histology indicates that specimens 2–6 were 2 years old at time of death, whereas specimen 1 was 3 years old. Scale bar is 5 cm. Figure 1: Cluster of six juvenile Psittacosaurus from the Lower Cretaceous of China. The cluster (IVPP V14341), shown in a photograph ( a ) and interpretive drawing ( b ), contains six aligned juvenile specimens of P. lujiatunensis . Bone histology indicates that specimens 2–6 were 2 years old at time of death, whereas specimen 1 was 3 years old. Scale bar is 5 cm. Full size image Limb allometry Length measurements from P. lujiatunensis long bones demonstrate that the humerus, radius and ulna are negatively allometric relative to the femur, with allometric coefficients of 0.89, 0.72 and 0.78, respectively ( Fig. 2 , Table 1 , Supplementary Table S2 ). The growth of the tibia and fibula relative to the femur is statistically distinguishable from isometry, but the coefficients (0.97 and 0.94, respectively; Fig. 2 , Table 1 , Supplementary Table S2 ) indicate only minimal negative allometry. The tibia remained slightly longer than the femur (averaging 110% of femoral length across the entire sample) throughout ontogeny. The forelimb became shorter relative to the hindlimb over the ontogeny of P. lujiatunensis ( Fig. 3 ), the allometric coefficient of forelimb length relative to hindlimb length being 0.83 ( Table 1 , Supplementary Table S2 ). In the three hatchling (<1 year old) individuals the forelimb-to-hindlimb ratio (the ratio of the combined length of the humerus and radius to that of the femur and tibia) averaged 0.84. The ratio averaged 0.70 in 1 year olds, but thereafter decreased gradually and steadily to an average of 0.61 in 7 year olds. The single 10-year-old specimen had an anomalously large ratio of 0.66, suggesting unusual proportions. The anomaly might be interpreted to support the original referral of this individual to H. houi [17] , but other aspects of this specimen’s morphology make a strong case for assigning it to P. lujiatunensis [5] , [16] . 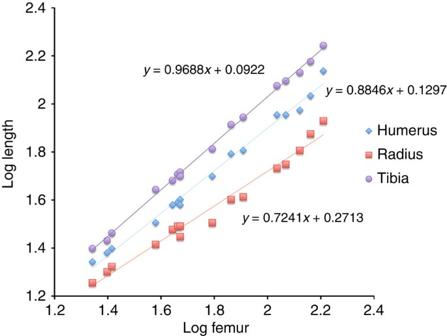Figure 2: Allometry in the appendicular skeleton ofPsittacosaurus. Allometric coefficients for ontogenetic growth inP. lujiatunensiscorrespond to slope values from a linear regression analysis of the lengths of the humerus, radius and tibia relative to that of the femur. Measurements of the ulna and fibula were very similar to those of the radius and tibia, respectively, so the ulna and fibula were omitted from the graph for the sake of clarity. Figure 2: Allometry in the appendicular skeleton of Psittacosaurus . Allometric coefficients for ontogenetic growth in P. lujiatunensis correspond to slope values from a linear regression analysis of the lengths of the humerus, radius and tibia relative to that of the femur. Measurements of the ulna and fibula were very similar to those of the radius and tibia, respectively, so the ulna and fibula were omitted from the graph for the sake of clarity. Full size image Table 1 Linear regressions of limb measurements in Psittacosaurus . 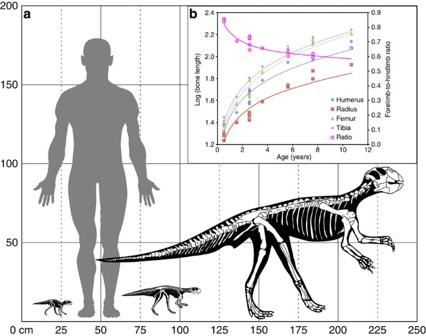Figure 3: Growth and postural change inPsittacosaurus. (a) Skeletal reconstructions of hatchling, juvenile and adult individuals ofP. lujiatunensisshowing inferred postural change, with 178-cm-tall man for scale. (b) Graph showing uneven length increases in various long bones, and changing values of the forelimb-to-hindlimb ratio, as a function of age in years. Forelimb elements increase in length more slowly than hindlimb elements, resulting in decreasing forelimb-to-hindlimb ratio and increasingly bipedal posture as growth continues. Long-bone measurements indicate the forelimb-to-hindlimb ratio changes most rapidly during early growth. Full size table Figure 3: Growth and postural change in Psittacosaurus . ( a ) Skeletal reconstructions of hatchling, juvenile and adult individuals of P. lujiatunensis showing inferred postural change, with 178-cm-tall man for scale. ( b ) Graph showing uneven length increases in various long bones, and changing values of the forelimb-to-hindlimb ratio, as a function of age in years. Forelimb elements increase in length more slowly than hindlimb elements, resulting in decreasing forelimb-to-hindlimb ratio and increasingly bipedal posture as growth continues. Long-bone measurements indicate the forelimb-to-hindlimb ratio changes most rapidly during early growth. Full size image Bone histology The thin sections of the 41 bones included in the histological analysis reveal many important details of vascular canal orientation and other aspects of microstructure. In all sections, the cortex is composed of fibrolamellar bone. The degree of vascularization is high in early growth, but appears to decrease abruptly beginning at the age of 4 or 5. Similarly, only primary osteons are present in younger individuals in the data set, but secondary osteons are visible in the long bones of all specimens that are at least 5 years old. Only the largest specimen shows evidence of remodelling of the secondary osteons. Forelimb and hindlimb bones show different patterns of canal orientation during ontogeny ( Fig. 4 ), although only limited information is available for the radius and ulna. Throughout most of ontogeny a combination of reticular and longitudinal canals is present in the humerus, the proportion of reticular canals being higher during the earlier half of growth and reaching a maximum in second-year bone (that is, bone deposited during the second year of life, between the first and second LAGs). In third-year bone both radial and reticular canals, as well as longitudinal ones, are present ( Fig. 5a ). These patterns suggest that bone was deposited rapidly during early growth of the humerus, but that the rate of deposition decreased in later ontogeny. For the radius and ulna, good histological evidence is available only for the first 3 years of growth, but bone formed during this period also shows a relatively high proportion of reticular canals in these elements. In the radius, third-year bone also contains radial canals, as in the humerus ( Fig. 5b ). The evidence based on canal orientation from the entire forelimb suggests rapid deposition of bone, consistent with a high level of vascularization during early growth. 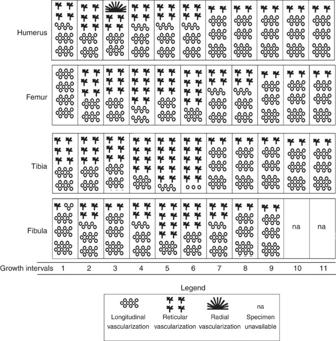Figure 4: Bone vascularization patterns during ontogeny inPsittacosaurus. The ontogenetic record of eachP. lujiatunensislong bone cross-section is divided into ‘growth intervals’ bounded by LAGs, so that bone of the first growth interval is ‘first-year bone’ lying within the first LAG. The icons for each growth interval of each bone depict the approximate relative abundances, as estimated from thin sections taken during our study, of the different vascular canal types present in bone formed during the growth interval in question. Format of diagram follows Erickson and Tumanova19except that their category of ‘radiating reticular vascularization’ is not used in our study. Figure 4: Bone vascularization patterns during ontogeny in Psittacosaurus . The ontogenetic record of each P. lujiatunensis long bone cross-section is divided into ‘growth intervals’ bounded by LAGs, so that bone of the first growth interval is ‘first-year bone’ lying within the first LAG. The icons for each growth interval of each bone depict the approximate relative abundances, as estimated from thin sections taken during our study, of the different vascular canal types present in bone formed during the growth interval in question. Format of diagram follows Erickson and Tumanova [19] except that their category of ‘radiating reticular vascularization’ is not used in our study. 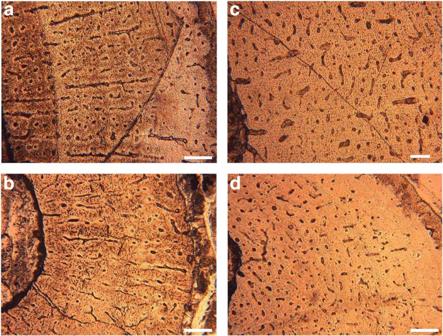Figure 5: Histological thin sections of juvenilePsittacosaurus. These sections are from two juvenile individuals ofP. lujiatunensispreserved in the same cluster (IVPP V14341), seen under normal light. Sections represent the humerus (a), radius (b), femur (c) and fibula (d), and were taken from the 2-year-old specimen IVPP V14341.6 (b) and the 3-year-old specimen IVPP V14341.1 (a,candd). Scale bar in each image is 200 μm. Full size image Figure 5: Histological thin sections of juvenile Psittacosaurus . These sections are from two juvenile individuals of P. lujiatunensis preserved in the same cluster (IVPP V14341), seen under normal light. Sections represent the humerus ( a ), radius ( b ), femur ( c ) and fibula ( d ), and were taken from the 2-year-old specimen IVPP V14341.6 ( b ) and the 3-year-old specimen IVPP V14341.1 ( a , c and d ). Scale bar in each image is 200 μm. Full size image Patterns of canal orientation in the hindlimb, however, are strikingly different. No hindlimb section shows radial canals at any stage of growth ( Figs 5 and 6 ), and the proportion of reticular as opposed to longitudinal canals is highest in bone formed during middle (approximately from ages three to six) rather than early ontogeny ( Fig. 5c ). The middle period of growth was therefore the time when bone was being deposited most rapidly in the hindlimb. 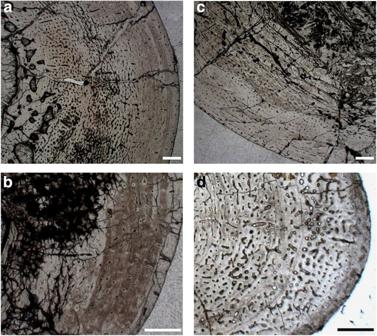Figure 6: Sections of subadult and adultPsittacosaurus. Mid-diaphyseal transverse sections represent the humerus (a), radius (b), femur (c) and fibula (d) ofP. lujiatunensis, and were taken from the 10-year-old individual IVPP V12617 (a,b), the 5-year-old individual IVPP V14749 (c), and the 7-year-old individual IVPP V18344 (d). Scale bar in each image is 500 μm. Figure 6: Sections of subadult and adult Psittacosaurus . Mid-diaphyseal transverse sections represent the humerus ( a ), radius ( b ), femur ( c ) and fibula ( d ) of P. lujiatunensis , and were taken from the 10-year-old individual IVPP V12617 ( a , b ), the 5-year-old individual IVPP V14749 ( c ), and the 7-year-old individual IVPP V18344 ( d ). Scale bar in each image is 500 μm. Full size image The observed changes in vascular canal orientation during the growth of particular long bones suggest shifts in the rate of bone deposition that may correlate with postural changes. This line of evidence indicates that deposition of bone was most rapid during early ontogeny in the forelimb elements. In the humerus, at least, growth appears to have slowed following deposition of the third LAG. In the hindlimb bones, by contrast, growth appears to have been most rapid during the fourth through sixth years of life. Unfortunately, histology does not provide a basis for directly comparing rates of bone deposition between the forelimb and the hindlimb. However, the fact that the forelimb appears to grow most rapidly during early ontogeny, whereas the hindlimb grows most rapidly during middle ontogeny, suggests a postural shift from quadrupedality to bipedality during the growth of P. lujiatunensis . In early ontogeny, the forelimb may have been growing rapidly, to maintain its proportional length and role in locomotion, whereas in middle ontogeny the simultaneous slowing of forelimb growth and acceleration of hindlimb growth may have caused the hindlimb to increase in relative length and assume primary responsibility for locomotion. However, the nature of the linkage between vascular canal orientation and the rate of length increase of a given bone requires further investigation, and the hypothesis that a postural shift took place in the growth of P. lujiatunensis requires further testing on the basis of limb bone measurements (see below). Histological patterns observed in this study ( Fig. 4 ) differ in some respects from those previously reported in a growth series of Psittacosaurus mongoliensis from the Lower Cretaceous of Mongolia [19] . The largest hindlimb bones (femur and tibia) in this growth series, representing individuals up to nine years old, show deposition of radially vascularized fibrolamellar bone along part of the mid-shaft circumference beginning at age 7. Other parts of the mid-shaft circumference have only reticular or even longitudinal vascularization. This indicates that local apposition rate differed greatly along the circumference of the bone, presumably reflecting osseous drift [19] . One possible explanation for the occurrence of radial vascularization is a postural shift ‘from bipedality to quadrupedality’ [19] , but this is unlikely given the strong evidence that adult individuals of Psittacosaurus were mainly bipedal (see below). The fitted growth curve for P. mongoliensis [19] indicates that at age 9 the largest sampled individuals had reached perhaps 80% of final body mass, a conclusion consist with the lack of an external fundamental system in any of the sampled bones. The largest histologically sampled individuals of P. mongoliensis thus appear to have been well short of final adult size and still within the exponential phase of growth [19] , perhaps indicating that the presence of radial canals in the hindlimb bones reflects normal growth along a sigmoid curve of mass versus age as in other dinosaurs including P. lujiatunensis [20] . However, the fact that the radial canals are limited to the hindlimb implies fast growth of the hindlimb relative to the forelimb at this stage of ontogeny, perhaps indicating a quadrupedal-to-bipedal postural shift like that inferred for P. lujiatunensis in the present study. However, radial canals were not observed in any of the hindlimb bones that we sectioned, suggesting that their occurrence in P. mongoliensis represents either a genuine difference in growth pattern between the two species or a result of pathology [19] . The largest P. mongoliensis femur sampled was 210 mm long, representing a 9-year-old animal that had still not reached maximal body size. By contrast, the largest known P. lujiatunensis femur measures 202 mm (ref. 20 ), and must have been close to final size because the largest femur sampled in the present study is only about 160 mm long but appears almost fully grown on the basis of histology. This femur represents an individual (IVPP V12617) that we consider to be 10 years old on histological grounds, although it was previously interpreted as a 6 year old based on femur size alone [20] . Femur length comparisons informed by histology suggest larger adult body size in P. mongoliensis , but inferred growth curves for the two species [19] , [20] show a considerably higher mass for P. lujiatunensis than for P. mongoliensis (38 kg in the former versus 25 kg in the latter). There are several possible solutions to this paradox, including the fact that the mass estimates used to construct the growth curves were based on circumference rather than length measurements [19] , [20] and could represent a difference in robustness between the two species, but distinguishing among the various possibilities will require an analysis directly comparing the two species in terms of both histology and skeletal proportions. We note, however, that both logistic growth curves extrapolate well beyond the available histological data, and we therefore prefer the direct histological and meristic evidence suggesting that P. mongoliensis grew to a larger final size than P. lujiatunensis . The greater inferred adult femur length of P. mongoliensis presumably indicates that the body mass of mature individuals was also greater in this species than in P. lujiatunensis , unless the two taxa were strikingly different in their proportions. We conclude that the histological evidence for a postural shift presented in this study for P. lujiatunensis is corroborated by histological evidence [20] in P. mongoliensis . In both cases, histology shows a differential change in bone apposition at mid-shaft, with the hindlimb bones speeding up growth relative to the forelimb bones. The specific changes in histology differ between the two species of Psittacosaurus , and the shift appears to have happened at a larger body size in P. mongoliensis than in P. lujiatunensis , consistent with the presumably larger final body size of the former. Psittacosaurus has been generally regarded as a habitual or obligate biped [6] , [7] , [8] , [10] , [11] , [12] , although the structure of the manus [6] , [7] and a few other skeletal features [21] have been interpreted as indicating some quadrupedal capability. A recent analysis of the distribution of osteological correlates of quadrupedality among ornithischians strongly favoured the view that Psittacosaurus was mainly bipedal [22] . Ornithischian quadrupeds typically possess a large anterolateral process on the ulna, hoof-like manual unguals, an everted dorsal edge of the ilium, a reduced fourth trochanter, and a femur that is longer than the tibia. In P. lujiatunensis specimens of any age the proximal end of the ulna bears only a small, laterally directed bulge, the dorsal edge of the ilium is narrow and non-everted, the fourth trochanter is large and pendant when preserved intact, and the tibia is slightly longer than the femur. Few well-preserved manual unguals are present in our sample. Available examples are shorter relative to their width than the pedal unguals, but are pointed rather than hoof-like. This suite of characters, which is shared with other very basal ceratopsians [22] , strongly suggests that P. lujiatensis was bipedal. However, this interpretation may only apply to adults. Ontogenetic changes in the various indicators of quadrupedality have not been investigated [22] , and it is uncertain how the features in question would be affected by an ontogenetic postural shift of the kind inferred for some dinosaurs. The forelimb-to-hindlimb ratio has traditionally been used as a postural indicator in dinosaurs [23] , with high ratios indicating quadrupedality. However, the utility of this metric in distinguishing quadrupeds from bipeds may be limited [22] . The ratio in subadult to adult P. lujiatunensis , as determined in this study (0.59–0.66), corresponds to the lower part of that reported by Maidment and Barrett [22] for eurypodan thyreophorans, even though other osteological indicators point clearly to bipedality for Psittacosaurus and quadrupedality for eurypodans. Similarly, the ancestral value of 0.67 reconstructed by Maidment and Barrett [22] for the unambiguously quadrupedal ceratopsids falls only just outside the range for subadult to adult P. lujiatunensis . There appears to be a range of values consistent with either bipedality or quadrupedality. However, the forelimb-to-hindlimb ratio is extremely high (averaging 0.84) in hatchlings of P. lujiatunensis , far exceeding values typical of eurypodans, ceratopsids and other quadrupedal dinosaurs [22] . The extreme values seen in hatchlings strongly suggest that they were essentially quadrupeds. This points to an ontogenetic shift along the continuum from quadrupedality to bipedality in the ontogeny of P. lujiatunensis , although the shift was not necessarily between obligate versions of the former and latter conditions. It is possible, for example, that hatchlings were primarily quadrupedal but resorted to bipedality at high speeds, whereas adults were quadrupedal only when moving very slowly. However, the proportionally long forelimbs of hatchlings, combined with the skeletal evidence for bipedality in adults, clearly implies that at least a limited postural shift took place. We envision the body of P. lujiatunensis as fundamentally suited to bipedality [22] . Hatchlings, however, were equipped with long forelimbs that could have been placed on the substrate when necessary to provide stability, particularly during slow locomotion. As an individual matured, its forelimb would have grown proportionally shorter, its balance would presumably have improved, and the forelimb would have contacted the substrate less often. Histology contributes to understanding of the ontogeny of posture in P. lujiatunensis in that counting LAGs makes it possible to relate changes in forelimb-to-hindlimb ratio to age in years, demonstrating that very high values were confined to specimens with less than one LAG. One-year-olds may have already been significantly less quadrupedal than hatchlings, and any subsequent changes were gradual. Growth patterns inferred from measurements of long bones can also be compared with patterns of bone deposition inferred from histology. The two lines of evidence agree, and reinforce each other, to the extent that both suggest a shift from quadrupedality to bipedality based on an increasing length discrepancy between the hindlimb and the forelimb over the course of ontogeny. However, histology also suggests that the shift occurred sometime after completion of the third year of growth, when forelimb growth accelerated and hindlimb growth was retarded, while measurements of long bones imply that the shift was at least initiated earlier based on rapid decrease in the forelimb-to-hindlimb ratio during early ontogeny. Furthermore, long-bone measurements do not appear to confirm the histological evidence for particularly rapid growth of the forelimb bones during early ontogeny, and particularly rapid growth of the hindlimb bones during middle ontogeny. It is likely that these discrepancies between histological evidence and limb bone measurements regarding growth in P. lujiatunensis are at least partly the result of inadequate sample size, and random variation in the limb proportions of the individuals in the data set. Although measurements of limb bones provide strong evidence for a shift towards greater bipedality, these data may be spread too thinly across ontogeny to reliably pinpoint when and how the shift took place. However, the discrepancies between histological and measurement-based inferences about growth also suggest that the relationship between vascular canal orientation and rate of increase in actual bone dimensions requires further investigation, and may be a particularly fruitful area for future research. The negative forelimb allometry that evidently characterized the ontogeny of P. lujiatunensis is comparable to that previously reported in the sauropodomorph dinosaur Massospondylus , which is inferred based on patterns of skeletal allometry to have been quadrupedal as a hatchling but to have shifted to a bipedal posture later in ontogeny [2] , [24] . Even hatchlings of at least some therizinosaurian theropods may have been preferentially quadrupedal, given the existence of embryos whose forelimbs are nearly equal in length to their hindlimbs [25] , although in the absence of preserved hatchlings this inference must be considered uncertain. An ontogenetic shift from quadrupedality to bipedality has also been inferred in the ornithopod Dryosaurus , based on changes in the femoral cross-sectional geometry during growth [26] . By contrast, the ornithopods Maiasaura and Iguanodon are inferred to have undergone a postural shift from juvenile bipedality to adult quadrupedality [3] , [4] . Our findings add to a growing body of evidence suggesting that ontogenetic quadrupedal-to-bipedal postural shifts were widespread in dinosaurs. Such shifts have now been inferred to have taken place in some members of at least two of the three major dinosaurian clades, Sauropodomorpha and Ornithischia. There is even a possible example of such a shift within the third clade, Theropoda, based on the elongate forelimbs that have been reported in therizinosaurian embryos [25] . However, the humerus measures 55–65% of the length of the femur in some theropod embryos, including oviraptorid [27] and troodontid [28] specimens, in striking contrast to the near-equality in length between the humerus and femur seen in the therizinosaurians [25] . It is clear that hatchlings were bipedal in some theropods, even if they were quadrupedal in at least some therizinosaurians. Selection acting on juveniles must have favoured bipedal hatchlings in some theropods and ornithopods, but quadrupedal hatchlings in other theropods, some ornithischians, and at least some sauropodomorphs. The possibility that basal members of all three major dinosaurian clades retained a quadrupedal hatchling stage is intriguing and cannot presently be excluded, but awaits further testing based on future discoveries. Similarly, the quadrupedal-to-bipedal shifts that occur in at least some taxa may recapitulate the evolutionary transition from quadrupedal basal archosaurs to bipedal avemetatarsalians that took place during the Early and Middle Triassic [29] , [30] , but this scenario will remain speculative until more information is available regarding the ontogeny of the early avemetatarsalian bipeds themselves. Our study highlights the benefits of considering histology alongside limb proportions and qualitative morphological features in studying the ontogeny of posture and locomotion in a fossil tetrapod. Counting LAGs makes it possible to roughly determine the age of each individual sampled, which provides a basis for determining the timing of changes in both limb bone measurements and patterns of vascular canal orientation. Measurements of limb bones for individuals of known ages can be used to build up a direct but discontinuous record of growth, defined as increase in bone dimensions, whereas the complementary record provided by vascular canal orientation and other histological features is indirect but continuous. Quantitative analysis of the link between histological indicators of bone growth and changes in the actual dimensions of long bones remains as an intriguing avenue for future research, and one that may eventually make it possible to use histology as a basis for more precise inferences about growth patterns and postural shifts. Histological sectioning Histological thin sections of long bones were made using standard techniques. Previous studies of dinosaur long-bone histology, as well as general principles of bone growth, indicate that a section taken at the middle of the shaft of a long bone is optimal for obtaining a maximally complete growth record from that bone [19] , [31] , [32] . This arises from the predominantly appositional growth of this part of the shaft, and the location of the neutral zone in this region [32] . Specimens were embedded in resin, and mid-shaft, diaphyseal transverse thin sections were cut using a diamond circular saw fitted with a diamond-tipped wafering blade. One surface of each section was smoothed with a wheel grinder/polisher, and then ground manually using grinding powder (600 grit) to produce a smooth texture ideal for gluing to a glass slide. The section was then cut to a thickness of about 250 μm with a diamond circular saw before being ground further to the desired final thickness of 50–80 μm, leaving the exposed surface of the section smooth. Each slide was then cleaned in a water-filled ultrasonic cleaner to remove microscopic grit, and finally capped with a glass cover slip. The completed thin sections were studied in normal and polarized light. Age determination The histological sections made it possible to estimate the age in years of each individual at the time of death, based on the typical pattern of formation of LAGs on an annual basis in dinosaur long bones. In sections that showed a small medullary cavity, the number of visible LAGs was taken to correspond approximately to the individual’s age in years, although it is unlikely that each LAG was formed exactly on the anniversary of hatching. Strictly speaking, the number of LAGs can be taken as a maximum bound on age in years, with a possible error of several months, but in this paper we use the phrase ‘ N -year-old individual’ to mean ‘individual in which N LAGs had formed’. However, the phenomenon of enlargement of the medullary cavity during growth introduced a well-understood complication [33] , in that such enlargement occurs through internal resorption of the bone cortex that may eliminate LAGs beginning with the innermost. To avoid underestimating ages as a result of this type of erosion, we used smaller examples of the bone in question as a reference point. The section being evaluated was graphically superimposed on equivalently orientated sections from smaller bones, and any LAG from the smaller bone that was entirely overlapped by the medullary cavity of the larger bone was assumed to be missing in the latter. For example, only two LAGs are visible in the tibia of IVPP V14341.1, but superimposing the section of this tibia on tibial sections from smaller individuals indicated that the medullary cavity of IVPP V14341.1 was large enough to have subsumed the first LAG formed during growth of the tibia ( Supplementary Figs S3–4 ). Accordingly, the LAGs visible in this specimen were identified as the second and third, rather than the first and second, and the specimen was identified as a 3 years old. Similarly, it can be inferred that the three innermost LAGs were obliterated by medullary cavity expansion in the humerus of the adult specimen IVPP V12617 ( Fig. 7 ). 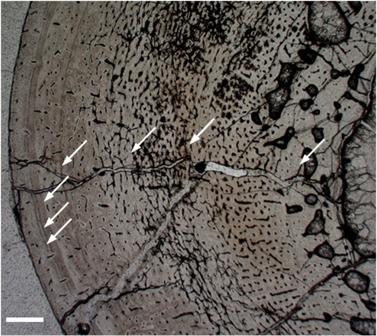Figure 7: Humeral section of adultPsittacosaurus. White arrows indicate the seven visible LAGs in the humerus of this specimen ofP. lujiatunensis(IVPP V12617), seen under normal light. The diameter of the medullary cavity is 5.8 mm, exceeding the diameter of the third year LAG in the humerus of IVPP V14341.1 (5.3 mm). This indicates that the three innermost LAGs have been obliterated by the medullary cavity in the larger humerus, and that IVPP V12617 is a 10-year-old individual rather than a 7-year-old. Superposition of cross-sections through the two humeri confirms graphically that three LAGs are missing in the larger one. Scale bar is 500 μm. Figure 7: Humeral section of adult Psittacosaurus. White arrows indicate the seven visible LAGs in the humerus of this specimen of P. lujiatunensis (IVPP V12617), seen under normal light. The diameter of the medullary cavity is 5.8 mm, exceeding the diameter of the third year LAG in the humerus of IVPP V14341.1 (5.3 mm). This indicates that the three innermost LAGs have been obliterated by the medullary cavity in the larger humerus, and that IVPP V12617 is a 10-year-old individual rather than a 7-year-old. Superposition of cross-sections through the two humeri confirms graphically that three LAGs are missing in the larger one. Scale bar is 500 μm. Full size image Vascular canal orientation We classified vascular canals visible in our thin sections as longitudinal, radial or reticular [33] , and noted which canal types were present in each growth interval (that is, interval bounded by LAGs) in each section. The relative numbers of the different canal types present were visually estimated. Provided that the medullary cavity had not expanded enough to destroy part of the record, a specimen with N LAGs could provide information about the vascularity of bone formed during the first year of growth (first-year bone), and bone formed during all subsequent years up to N+1. For example, a specimen with two LAGs could provide information about the vascularity of first year, second year and third year bone. Given that reticular and particularly radial canals are associated with relatively rapid deposition of bone, based on evidence from living birds [34] , their presence was taken as an indication of rapid deposition in P. lujiatunensis . Limb bone allometry Coefficients of allometry were calculated for the lengths of the humerus, radius, ulna, tibia and fibula relative to that of the femur, and for forelimb (humerus+radius) length relative to hindlimb (femur+tibia) length. The length measurements were log-transformed and then saved as a.txt file that could be read by the computer program R (R Development Core Team, 2008). As in previous work [24] , the slope of the regression line on a bivariate plot of the lengths of two bones or limbs was interpreted as the allometric coefficient of length for one bone or limb relative to the other. Linear regressions were carried out in R, using the lm command. In all cases the 95% confidence interval for the slope excluded the isometric value of 1, indicating statistically significant negative (for coefficients <1) or positive (for coefficients >1) allometry relative to the femur or hindlimb. How to cite this article: Zhao, Q. et al. Histology and postural change during the growth of the ceratopsian dinosaur Psittacosaurus lujiatunensis . Nat. Commun. 4:2079 doi: 10.1038/ncomms3079 (2013).